Copper-catalyzed carbo-difluoromethylation of alkenes via radical relay Organic molecules that contain alkyl-difluoromethyl moieties have received increased attention in medicinal chemistry, but their synthesis in a modular and late-stage fashion remains challenging. We report herein an efficient copper-catalyzed radical relay approach for the carbo-difluoromethylation of alkenes. This approach simultaneously introduces CF 2 H groups along with complex alkyl or aryl groups into alkenes with regioselectivity opposite to traditional CF 2 H radical addition. We demonstrate a broad substrate scope and a wide functional group compatibility. This scalable protocol is applied to the late-stage functionalization of complex molecules and the synthesis of CF 2 H analogues of bioactive molecules. Mechanistic studies and density functional theory calculations suggest a unique ligand effect on the reactivity of the Cu-CF 2 H species. The rapid construction of fluorine-containing organic molecules has attracted considerable attention, owing to the special ability of a fluorine atom or a fluoroalkyl group to modulate the metabolic stability, lipophilicity, and membrane permeability of a drug candidate [1] , [2] , [3] , [4] , [5] . Among the many fluorine-containing groups, the difluoromethyl group (CF 2 H) is drawing ever-increasing attention due its unique ability to act as a possible lipophilic hydrogen bond donor and thus a potential bioisostere for hydroxyl, amino, or thiol groups [6] , [7] , [8] , [9] , [10] , [11] , [12] , [13] , [14] , [15] , [16] , [17] , [18] , [19] , [20] . It is not surprising, therefore, that pharmaceutical companies began to investigate CF 2 H-containing lead compounds and intense research has been focused on the development of efficient methods for the installation of CF 2 H groups. Over the past decade, significant progress has been made in the subject of difluoromethylation of arenes [21] , [22] , [23] , [24] , [25] , [26] , [27] , [28] , [29] , [30] , [31] , [32] , [33] , [34] , [35] , [36] , [37] . However, analogous methods for the synthesis of alkyl-difluoromethanes have lagged behind, despite the high pharmaceutical relevance of these molecules (Fig. 1a ). Fig. 1: Copper-catalyzed carbo-difluoromethylation of alkenes could enable modular synthesis of complex alkyl-difluoromethanes. a Complex alkyl-difluoromethanes as pharmaceuticals. b A state-of-the-art method for the synthesis of alkyl-difluoromethanes. c Copper-catalyzed carbo-difluoromethylaton of alkenes. Full size image Vicinal carbo-difluoromethylation of widely available alkenes, which results in the simultaneous formation of an alkyl–CF 2 H bond and a C–C bond, is an attractive, efficient, and potentially modular method for the synthesis of complex alkyl-difluoromethanes. Elegant work has recently been conducted by Dolbier [38] , Qing [39] , Xiao [40] , Gouverneur [41] , Zhang [42] , Chu [43] , and others [6] , [44] for the difluoromethylation of alkenes by harnessing the reactivity of an in situ generated difluoromethyl or difluoroalkyl radical. Although these state-of-the-art methods allow for the rapid difluoromethyl-functionalization of alkenes, nonetheless, in these reactions the CF 2 H group is generally attached to the terminal side of the alkenes, as dictated by the CF 2 H radical addition to the less sterically hindered site. In addition, the groups installed to the remaining site of the alkenes are limited to either hydrogen atoms or other simple functional groups (Fig. 1b ). Therefore, an alternative strategy allowing for the introduction of a diverse range of groups onto alkenes with complementary regioselectivity would open an avenue for the discovery of CF 2 H-pharmaceuticals. Our group has recently demonstrated that copper can catalyze the efficient transfer of a CF 2 H group to an alkyl radical. This mode of CF 2 H transfer allowed us to develop the first decarboxylative [45] , deaminative [46] and benzylic C–H difluoromethylation reactions [47] . These reactions proceed via copper-catalyzed generation of an alkyl radical which can be trapped by a [Cu II -CF 2 H] intermediate and go through reductive elimination to generate the desired alkyl-difluoromethane. We recently wondered whether this Cu/CF 2 H system could be applied to the difunctionalization of alkenes by intercepting the radical intermediate with a suitable alkene to form a relayed radical [48] , [49] , [50] , [51] , [52] , [53] , [54] . Subsequent copper-CF 2 H trapping/reductive elimination of the relayed radical could then allow for the carbo-difluoromethylation of the alkene. We anticipated that, by varying the radical precursors and alkene partners, this approach could enable the synthesis of complex alkyl-difluoromethanes in a modular fashion (Fig. 1c ). A plausible mechanism for the proposed carbo-difluoromethylation reaction is shown in Fig. 2 . A transmetalation of a copper(I) catalyst 1 with a [Zn II -CF 2 H] reagent is expected afford a reactive [Cu I -CF 2 H] species 3 [23] , [26] , [28] , [33] , [34] , [55] , which should readily reduce a suitable alkyl or aryl electrophile 4 , to form a carbon-centered radical 5 . This radical species would then undergo a radical addition to an alkene 6 , to generate the resultant relayed radical 7 . The subsequent radical recombination of 7 with the [Cu II -CF 2 H] complex 8 could generate a formal Cu III intermediate 9 [56] , which undergoes reductive elimination to forge the desired alkyl-difluoromethane product 10 . This reductive elimination step regenerates the Cu I catalyst and closes the catalytic cycle [57] , [58] . We recognized that a critical factor to the success of this reaction would be the selective addition of the carbon-centered radical 5 to the alkenes in lieu of direct recombination to the [Cu II -CF 2 H] species. We expected that controlling the rates of radical recombination to the copper catalyst would be necessary to achieve the desired transformation. It is noteworthy that although difunctionalization of alkenes via a copper-catalyzed radical relay process—the concept of which was first conveyed by Liu and Stahl [59] —has been reported [60] , [61] , [62] , [63] , the simultaneous formation of two Csp 3 –Csp 3 bonds via this process remains rare [64] . Fig. 2: Proposed catalytic cycle for the copper-catalyzed carbo-difluoromethylation of alkenes. The proposed mechanism involves the single electron transfer (SET) from a [Cu-CF 2 H] species to an electrophile to form a carbon-centered radical, which reacts with an alkene to afford a relayed radical. The relayed radical reacts with a [Cu II -CF 2 H] species to form the difluoromethylated product. Full size image In this work, we report a copper-catalyzed carbo-difluoromethylation reaction that can simultaneously introduce CF 2 H groups and complex alkyl or aryl groups into alkenes with the regioselectivity opposite to traditional CF 2 H radical chemistry. Difluoromethyl-alkylation of alkenes Based on our previous work on the decarboxylative difluoromethylation of redox-active esters (RAEs), we first questioned whether an alkyl radical generated in situ from RAEs could participate in this reaction, allowing for the development of the difluoromethyl-alkylation of alkenes. Thus, we began our studies with the RAE of tetrahydropyran-4-carboxylic acid 11 as the alkyl electrophile, with styrene as the alkene partner. Different copper salts, ligands, and CF 2 H sources were evaluated (Fig. 3 ). To our delight, we found that the use of CuCl as the catalyst, along with (terpy)Zn(CF 2 H) 2 (terpy = 2,2ʹ:6ʹ,2ʺ-terpyridine) as the CF 2 H source, generated via mixing terpy and (DMPU) 2 Zn(CF 2 H) 2 in situ, the product 12 could be formed in a 76% yield in dimethyl sulfoxide (DMSO) at room temperature (r.t.) (entry 1). The formation of 12 represents a rare example of the simultaneous formation of two Csp 3 –Csp 3 bonds via a copper-catalyzed radical relay process. In addition, the side product 12a , derived from the direct trapping of the alkyl radical by the [Cu II -CF 2 H] species, was formed in a 11% yield under the optimized conditions. Intriguingly, the ligand used in the reactions plays a vital role in this transformation. No desired products were formed when styrene was added to our previously established decarboxylative difluoromethylation conditions, in which 2,2ʹ-bipyridine (bpy) was used as the ligand (entry 2). 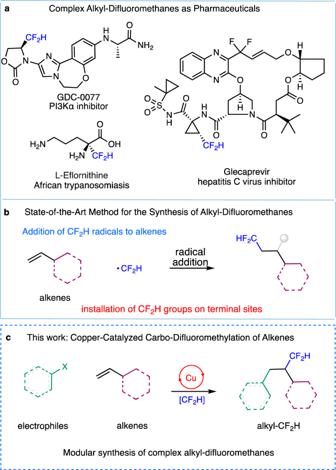Fig. 1: Copper-catalyzed carbo-difluoromethylation of alkenes could enable modular synthesis of complex alkyl-difluoromethanes. aComplex alkyl-difluoromethanes as pharmaceuticals.bA state-of-the-art method for the synthesis of alkyl-difluoromethanes.cCopper-catalyzed carbo-difluoromethylaton of alkenes. Other bidentate ligands provided essentially no products (Supplementary Table 1 ) and lower yields were observed when other substituted terpy ligands were used instead of terpy (entry 3). No desired product was formed when (DMPU) 2 Zn(CF 2 H) 2 was used as the difluoromethyl source without the addition of terpy (entry 4). Trace amounts of products were formed when the analogous N-hydroxyphthalimide (NHPI) ester was used (entry 5). 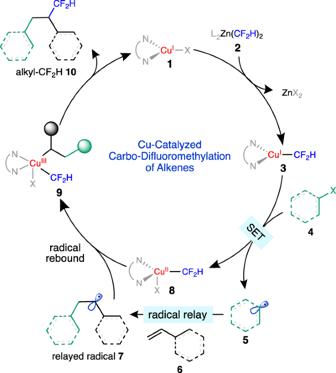Fig. 2: Proposed catalytic cycle for the copper-catalyzed carbo-difluoromethylation of alkenes. The proposed mechanism involves the single electron transfer (SET) from a [Cu-CF2H] species to an electrophile to form a carbon-centered radical, which reacts with an alkene to afford a relayed radical. The relayed radical reacts with a [CuII-CF2H] species to form the difluoromethylated product. Different copper(I) and copper(II) salts could also be used (entries 6 and 7 and Supplementary Table 2 ), albeit with lower efficiency. Varying the amounts of (terpy)Zn(CF 2 H) 2 and increasing the reaction temperature led to diminished yields (entries 8–10). The styrene loading can be reduced to 2 equiv., yet attaining a synthetically useful yield (entry 11). No difluoromethylated products were formed when the reactions were conducted in the absence of copper catalysts (entry 12). This reaction could also be set up outside of the glovebox without affecting the yield (entry 13 and Supplementary Method 1 ). Fig. 3: Optimization of the copper-catalyzed difluoromethyl-alkylation of alkenes. Reactions were conducted with 11 (0.1 mmol, 1.0 equiv. ), styrene (0.3 mmol, 3.0 equiv. ), (terpy)Zn(CF 2 H) 2 (0.08 mmol, 0.8 equiv.) and CuCl (30 mol%) in DMSO (0.4 mL). (terpy)Zn(CF 2 H) 2 was formed in situ by pre-mixing (DMPU) 2 Zn(CF 2 H) 2 and terpy in DMSO. Yields were determined by 19 F NMR using 1-fluoro-3-nitrobenzene as the internal standard. terpy, 2,2ʹ;6ʹ,2ʺ-terpyridine; DMSO, dimethyl sulfoxide; NHPI, N-hydroxyphthalimide; DMPU, N , N ′-Dimethylpropyleneurea. Full size image With the optimized conditions in hand, we began to evaluate the scope of vinyl arenes (Fig. 4 ). A wide range of electron-withdrawing, electron-donating, and electron-neutral functional groups could be tolerated on the aryl rings ( 12–28 ). The reactivity was not hindered by ortho substitutions on the vinyl arene ring ( 16 ). A basic tertiary amine group, which is usually problematic in transition metal catalysis, was tolerated ( 18 ). The compatibility with an aryl chloride ( 22 ) provides the basis for the further synthetic manipulation of the difluoromethylated products. This protocol allowed for the efficient installation of nitrogen- and oxygen-containing heterocycles, including benzofuran ( 26 ), unprotected indole ring ( 27 ), and pyrazole ( 28 ), which are ubiquitous in pharmaceuticals, into alkyl-CF 2 H moieties in good yields. It is worth noting that the excess vinyl arenes could be recovered with excellent mass balance (Supplementary Method 1 ). Fig. 4: Copper-catalyzed difluoromethyl-alkylation of alkenes. Reactions were run with 0.25 mmol of RAEs, 0.75 mmol of alkenes (3.0 equiv. ), 0.2 mmol of (terpy)Zn(CF 2 H) 2 (0.8 equiv. ), and CuCl (30 mol%) in 1 mL of DMSO at r.t., isolated yields based on RAEs. a Reaction performed under modified conditions (Supplementary Method 5 ). terpy, 2,2ʹ;6ʹ,2ʺ-terpyridine; DMSO, dimethyl sulfoxide. Full size image We next turned our attention to the scope of carboxylic acids for this protocol. To our delight, this reaction was amenable to a wide range of secondary and tertiary carboxylic acids. RAEs derived from secondary carboxylic acids appended to a variety of four-, five-, six-, or seven-membered rings, paired with different functional groups could be successfully employed to deliver the desired products in good to excellent yields ( 29–45 ). Oxygen-containing saturated heterocycles, such as tetrahydrofuran ( 36, 37 ) and tetrahydropyran ( 38 ), were successfully employed in this reaction. Carboxylic acids derived from piperidine, one of the most prevalent ring systems found in drug molecules [65] , could undergo efficient difluoromethylation ( 40–43 ). Nitrogen-containing heterocycles, which are core structures in drug synthesis, including pyrimidine ( 40, 42 ) and pyridine ( 41 ), were all accommodated in this protocol. Two bicyclic and spirocyclic carboxylic acids were successfully converted to the desired products with good efficiency ( 44, 45 ). Furthermore, acyclic and cyclic tertiary carboxylic acids could undergo the radical relay pathway to give the desired products in good yields ( 46–51 ). Moderate yields were observed when a phenyl group was connected to the tertiary carboxylic acid ( 49 ), likely due to the lower reactivity of a tertiary benzylic radical. In addition to RAEs, activated alkyl bromides ( 52, 53 ) and an alkyl pyridinium salt ( 37 ) were found to participate readily in this reaction, providing the corresponding alkyl-CF 2 H products in good yields. Poor yields were observed when the RAEs of primary carboxylic acids were employed in the reactions and the decarboxylative difluoromethylated products were found to be the dominant products. To further showcase the synthetic utility of this carbo-difluoromethylation protocol for the construction of complex alkyl-difluoromethanes, we sought to apply it to the late-stage modification of pharmaceuticals and natural products. Modification of a lipid regulating agent, gemfibrozil, afforded the desired alkyl-difluoromethane 54 in a 62% yield. Furthermore, we undertook the rapid functionalization of two complex steroidal acids, glycyrrhetinic acid and oleanolic acid, both of which could be converted to the corresponding difluoromethylated products in synthetically useful yields ( 55–57 ). The fact that unprotected hydroxyl groups could be well tolerated in these transformations further highlighted the mild conditions of this copper-catalyzed process. Given the ubiquity of carboxylic acids and alkenes, we expect that this protocol will find wide application in the field of medicinal chemistry for the synthesis of complex CF 2 H-containing pharmaceuticals in a modular fashion. Difluoromethyl-arylation of alkenes Having demonstrated that in situ generated alkyl radicals can participate in this carbo-difluoromethylation protocol, we further questioned whether aryl radicals could also be engaged in this reaction, allowing for the simultaneous introduction of an aryl and a CF 2 H group to various alkenes. A possible source for aryl radicals could be aryl diazonium salts, which are readily prepared from various anilines. We reasoned that an aryl diazonium salt could undergo a homolytic bond cleavage in the presence of a reactive [Cu I -CF 2 H] species, forming an aryl radical [34] , which could react with an alkene via the Meerwein-type arylation pathway. The relayed radical could be trapped by a [Cu II -CF 2 H] species, forming the desired difluoromethylated product via the radical recombination/reductive elimination pathway. It is noteworthy that although the Meerwein arylation reaction, which was originally reported by Hans Meerwein in 1939 [66] , has been developed as a useful method for the functionalization of alkenes [67] , the interception of the relayed radical by a copper catalyst for the construction of a C–C bond remains elusive. We have found that in the presence of [Cu(CH 3 CN) 4 ]BF 4 (20 mol%) as the catalyst, terpy (20 mol%) as the ligand and (DMPU) 2 Zn(CF 2 H) 2 as the difluoromethyl source, various aryl diazonium salts could undergo efficient difluoromethylation with different alkenes as the radical acceptors (Fig. 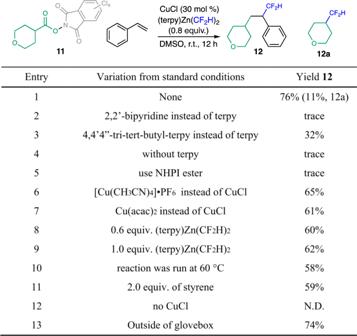Fig. 3: Optimization of the copper-catalyzed difluoromethyl-alkylation of alkenes. Reactions were conducted with11(0.1 mmol, 1.0 equiv.), styrene (0.3 mmol, 3.0 equiv.), (terpy)Zn(CF2H)2(0.08 mmol, 0.8 equiv.) and CuCl (30 mol%) in DMSO (0.4 mL). (terpy)Zn(CF2H)2was formed in situ by pre-mixing (DMPU)2Zn(CF2H)2and terpy in DMSO. Yields were determined by19F NMR using 1-fluoro-3-nitrobenzene as the internal standard. terpy, 2,2ʹ;6ʹ,2ʺ-terpyridine; DMSO, dimethyl sulfoxide; NHPI, N-hydroxyphthalimide; DMPU,N,N′-Dimethylpropyleneurea. 5 and see Supplementary Table 3 for optimization details). Aryl diazonium salts bearing electron-withdrawing or electron-donating groups reacted efficiently with vinyl arenes, affording the corresponding difluoromethylated products in good yields. Functional groups including halides ( 61–63 ), esters ( 64 ), ketones ( 68 ), and acetals ( 68 ) were well tolerated in these transformations. Ortho substitutions of the aryl diazonium salts did not hinder the reactivity ( 63 ). Aryl diazonium salts bearing heterocycles, such as dioxane ( 67 ), coumarin ( 69 ), and thioazole ( 70, 71 ), along with a heteroaryl diazonium salt ( 72 ) afforded the desired difluoromethylated products albeit in moderate yields. In addition to styrenes, other alkenes including acrylonitrile and methyl acrylate, could also be engaged in this difluoromethyl-arylation reaction, allowing for the rapid synthesis α-CF 2 H nitriles and α-CF 2 H esters ( 73–82 ). In addition, the difluoromethyl-arylation of acrylonitrile could also be conducted on a large scale. Without any modification of the standard conditions, the gram-scale synthesis of 76 could be produced in a similar yield to that obtained on a 0.25 mmol scale. Given the diverse reactivities of cyanide groups and ester groups, we expected that α-CF 2 H nitriles and α-CF 2 H esters could serve as highly useful building blocks for the preparation of other CF 2 H-containing moieties. For example, the treatment of an α-CF 2 H nitrile 76 with an alkaline solution of H 2 O 2 afforded an α-CF 2 H amide 83 in an 80% yield, while the reduction of 81 with diisobutylaluminium hydride (DIBAL-H) allowed for the synthesis of a β-CF 2 H alcohol 84 in an 85% yield. Fig. 5: Copper-catalyzed difluoromethyl-arylation of alkenes. Reactions were run with 0.25 mmol of aryl diazonium salts (1.0 equiv. ), 0.75 mmol of alkenes (3.0 equiv. ), 0.2 mmol of (DMPU) 2 Zn(CF 2 H) 2 (0.8 equiv. ), CuCl (20 mol%), and terpy (20 mol%) in 1 mL of DMSO at r.t., isolated yields. a See Supplementary Method 1 for detailed conditions. terpy, 2,2ʹ;6ʹ,2ʺ-terpyridine; DMSO, dimethyl sulfoxide. Full size image The synthetic utility of this difluoromethyl-arylation reaction has been further highlighted by the rapid synthesis of the CF 2 H analogue of combretastatin, 85 , in a 45% yield. Combretastatin and its derivatives are potent vascular targeting agents and are undergoing various clinical trials for treating different cancers [68] . Considering the known ability of a CF 2 H group to act as a bioisostere of a hydroxyl group, 85 could potentially be a metabolically stable analogue of combretastatin. Mechanistic studies Mechanistic studies were conducted to shed light on these carbo-difluoromethylation reactions (Fig. 6 ). In our previously reported decarboxylative difluoromethylation reactions, bpy was found to be the optimal ligand [45] , but the tridendate ligand, terpy, was uniquely effective for the current system. We were intrigued by the dramatic difference of the difluoromethylation reactivity with difference ligands. Mechanistic understanding of the effect of ligands on the difluoromethylation reactivity is vital for the development of other alkyl-CF 2 H bond-forming reactions and could shed light on copper-catalyzed C–C bond-forming reactions that involve alkyl radicals as intermediates. Fig. 6: Mechanistic studies. a Dimerization of the relayed radical with bpy as the ligand. b Effect of ligands on the decarboxylative difluoromethylation reactions. c Radical clock experiments. terpy, 2,2ʹ;6ʹ,2ʹʹ-terpyridine; bpy, 2,2ʹ-bipyridine; DMSO, dimethyl sulfoxide. Full size image When the carbo-difluoromethylation reaction of 86 was conducted with bpy as the ligand, trace amount of the desired product 87 was observed. Analysis of the reaction mixture by GC/MS showed that the dimerization of the relayed radical ( 88 ) was a major competing pathway (Fig. 6a and Supplementary Figs. 11 – 12 ). We hypothesized that the reason for this dramatic difference in reactivity with different ligand is that the relayed radical, a secondary benzylic radical, could smoothly react with the [(terpy)Cu II CF 2 H] intermediate but could not be efficiently trapped by a [(bpy)Cu II CF 2 H] species. 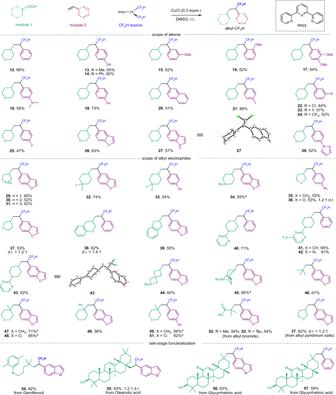Fig. 4: Copper-catalyzed difluoromethyl-alkylation of alkenes. Reactions were run with 0.25 mmol of RAEs, 0.75 mmol of alkenes (3.0 equiv.), 0.2 mmol of (terpy)Zn(CF2H)2(0.8 equiv.), and CuCl (30 mol%) in 1 mL of DMSO at r.t., isolated yields based on RAEs.aReaction performed under modified conditions (Supplementary Method5). terpy, 2,2ʹ;6ʹ,2ʺ-terpyridine; DMSO, dimethyl sulfoxide. Several additional experimental results further support this hypothesis. When a RAE derived from a secondary benzylic carboxylic acid, 89 , was subjected to the standard decarboxylative difluoromethylation conditions, trace amount of the difluoromethylated product 90 was detected with bpy as the ligand, a phenomenon we observed in our previous studies [45] . On the contrary, a nearly quantitative yield was observed for the formation of 90 when terpy was used as the ligand. Similarly, the RAE derived from an acyclic secondary carboxylic acid 91 could undergo efficient decarboxylative difluoromethylation with terpy as the ligand, forming 92 as the major product, while a poor reactivity was observed with a bpy ligand under otherwise identical conditions (Fig. 6b ). More importantly, in both cases, the dimerization of the secondary alkyl radicals was the competing reaction when bpy was used as the ligand (Supplementary Figs. 5 – 10 ). To take into account of an alternative possibility that this ligand effect is due to the differences in reactivity of the [Cu I -CF 2 H] species to undergo a single electron transfer event, we conducted the decarboxylative difluoromethylation of a radical clock substrate 93 ( Fig. 6c ). Direct decarboxylative difluoromethylation of 93 with either terpy or bpy as ligands under otherwise identical conditions both afforded the ring-opened product 94 in high yields along with trace amounts of the unrearranged product 95 . Although further experiments are necessary for the detailed comparison of the reactivity of different [Cu I -CF 2 H] species, these results support that both [(terpy)Cu I -CF 2 H] and [(bpy)Cu I -CF 2 H] species were reactive enough to undergo the single electron transfer events with the RAE 93 to generate the corresponding benzylic radical, which rearranged to a primary alkyl radical, affording 94 as the major product. The high yields of 94 with either ligand could be explained by the small steric interaction when a primary radical reacts with the [Cu II -CF 2 H] species. DFT calculation on the effect of ligands Our mechanistic studies suggest that acyclic secondary alkyl radicals could be more efficiently trapped by the [Cu II -CF 2 H] species coordinated to a terpy ligand. To better understand this ligand effect, we performed DFT calculations to probe the reaction between a secondary benzylic radical and the [Cu II -CF 2 H] species bound with a bpy or a terpy ligand (Fig. 7 ). Our previous DFT calculations [69] and Cook’s work [70] on the trifluoromethylation of benzylic C–H bonds have both indicated that the benzylic radical could recombine with a four-coordinate [(bpy)Cu II (CF 3 ) 2 ] species to form a five-coordinate high-valent copper(III) intermediate, [(bpy)Cu III (CF 3 ) 2 (benzyl)], which reductively eliminates to form the trifluoromethylated product. Very recently, the Shen group has successfully characterized the putative five-coordinate copper(III) complex, [(bpy)Cu III (CF 3 ) 2 (Me)], which could undergo C–CF 3 bond-forming reductive elimination to form 1,1,1-trifluoroethane [58] . These precedents suggest that Csp 3 -fluoroalkyl bond-forming reductive elimination would most likely occur on five-coordinate copper(III) complexes. Fig. 7: Energy profile of the reactions between a secondary benzylic radical with [Cu II -CF 2 H] species. a Energy profile of the reactions between a secondary benzylic radical with [(terpy)Cu II (CF 2 H)] species, b Energy profile of the reactions between a secondary benzylic radical with [(bpy)Cu II (CF 2 H) 2 ] species. Rad, benzylic radical; terpy, 2,2ʹ;6ʹ,2ʺ-terpyridine; bpy, 2,2ʹ-bipyridine; TS, transition state; TSre, transition state for reductive elimination; rel. G, relative Gibbs free energy. Full size image With this background in mind, we reasoned that when bpy was used as the ligand for the difluoromethylation reaction, a benzylic radical would react with a four-coordinate copper(II) intermediate which bound to two CF 2 H groups, [(bpy)Cu II (CF 2 H) 2 ] ( Cu-2 , Fig. 7 ), to form a five-coordinate copper(III) complex ( Cu-2A ), which reductively eliminated to form the difluoromethylated product. On the contrary, when the tridentate ligand, terpy, bound with the copper center, the four-coordinate copper(II) could only attach to one CF 2 H group ( Cu-1 ). The recombination of the benzylic radical with Cu-1 could form the five-coordinate high-valent copper(III) complex ( Cu-1A ), with only one CF 2 H bonding to the copper center. Interestingly, our DFT calculation found that the formation of the high-valent Cu III species ( Cu-1A ) from the combination of a benzylic radical ( Rad ) with Cu-1 was a barrierless pathway. In contrast, the reaction between Rad with Cu-2 required a high activation energy (Δ G ‡ = 21.8 kcal/mol, TS2 ), suggesting that the combination of the secondary benzylic radical, Rad , with Cu-1 was a much more efficient process than its reaction with Cu-2 . It is noteworthy that Cu-2 was found to combine with a cyclohexyl radical via a barrierless pathway (Supplementary Fig. 13 ), consistent with our previous experimental results that the Cu/bpy system was effective for the decarboxylative difluoromethylation of the RAEs derived from cyclic secondary carboxylic acids. Moreover, our calculation results demonstrated that the C–CF 2 H bond-forming reductive elimination step also contributed to the effect of ligands. As shown in Fig. 7 , the reductive elimination of Cu-1A proceeded with a significantly lower activation energy (Δ G ‡ = 6.3 kcal/mol, TSre-1 ) than that of Cu-2A (Δ G ‡ = 18.1 kcal/mol, TSre-2 ). Overall, these DFT calculations suggest that the success of the tridentate ligand, terpy, in the carbo-difluoromethylation reactions was largely due to a rapid combination of the secondary benzylic radicals with the Cu II intermediates as well as the facile reductive elimination of the Cu III species, although other factors including the difference of the transmetalation rates could not be ruled out. In conclusion, we reported herein a carbo-difluoromethylation of alkenes via a copper-catalyzed radical relay strategy, complementing the well-established CF 2 H radical addition to alkenes. This transformation allows for the rapid installation of CF 2 H groups and a diverse range of alkyl and aryl groups onto various vinyl arenes and Michael acceptors. This protocol could enable the efficient construction of complex alkyl-difluoromethanes in a modular fashion and rapid evaluation of structure–activity relationships of potential CF 2 H-containig pharmaceuticals. Furthermore, the difluoromethyl-alkylation protocol represents a rare example of a copper-catalyzed radical relay process for the simultaneous construction of two Csp 3 –Csp 3 bonds, while the difluoromethyl-arylation reaction could open an avenue for the development of other Meerwein-type arylation reactions. Mechanistic studies indicated a previously unknown effect of ligands on the reactivity of the putative [Cu-CF 2 H] species, which may serve as a guide in selecting ligands in other copper-catalyzed reactions which involve alkyl radicals as the intermediates. 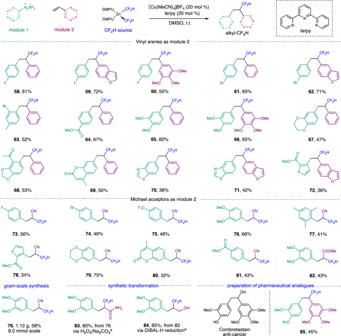Fig. 5: Copper-catalyzed difluoromethyl-arylation of alkenes. Reactions were run with 0.25 mmol of aryl diazonium salts (1.0 equiv.), 0.75 mmol of alkenes (3.0 equiv.), 0.2 mmol of (DMPU)2Zn(CF2H)2(0.8 equiv.), CuCl (20 mol%), and terpy (20 mol%) in 1 mL of DMSO at r.t., isolated yields.aSee Supplementary Method1for detailed conditions. terpy, 2,2ʹ;6ʹ,2ʺ-terpyridine; DMSO, dimethyl sulfoxide. 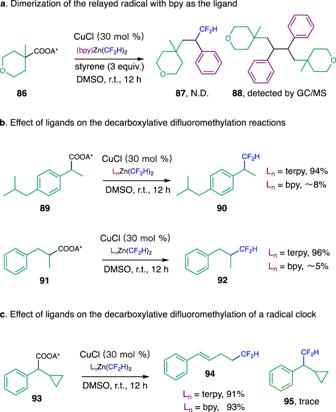Fig. 6: Mechanistic studies. aDimerization of the relayed radical with bpy as the ligand.bEffect of ligands on the decarboxylative difluoromethylation reactions.cRadical clock experiments. terpy, 2,2ʹ;6ʹ,2ʹʹ-terpyridine; bpy, 2,2ʹ-bipyridine; DMSO, dimethyl sulfoxide. 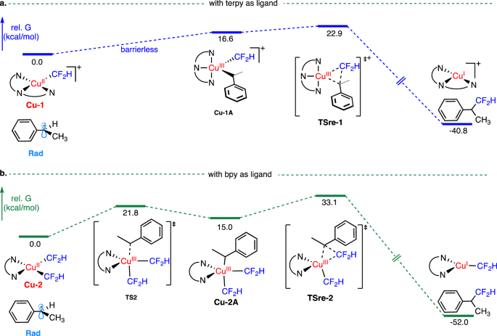Fig. 7: Energy profile of the reactions between a secondary benzylic radical with [CuII-CF2H] species. aEnergy profile of the reactions between a secondary benzylic radical with [(terpy)CuII(CF2H)] species,bEnergy profile of the reactions between a secondary benzylic radical with [(bpy)CuII(CF2H)2] species. Rad, benzylic radical; terpy, 2,2ʹ;6ʹ,2ʺ-terpyridine; bpy, 2,2ʹ-bipyridine; TS, transition state; TSre, transition state for reductive elimination; rel. G, relative Gibbs free energy. Further studies on the use of other electrophiles/radical acceptors and the asymmetric version of this reaction are currently ongoing in our laboratories. Difluoromethyl-alkylation of alkenes In a nitrogen-filled glovebox, to a 4 mL vial equipped with a stir bar was added terpyridine (0.8 equiv., 47 mg), (DMPU) 2 Zn(CF 2 H) 2 (0.8 equiv., 87 mg), and 800 μL DMSO. The resulting mixture was stirred at room temperature for 1 min to generate (terpy)Zn(CF 2 H) 2 in situ. A different 4 mL vial equipped with a stir bar was sequentially charged with CuCl (30 mol%, 7.5 mg), RAEs (0.25 mmol, 1.0 equiv. ), the DMSO solution of the in situ formed (terpy)Zn(CF 2 H) 2 , and alkene (0.75 mmol, 3.0 equiv.) in DMSO (200 μL). The resultant mixture was stirred at room temperature for 12 h. After the reaction was completed, the mixture was diluted with ethyl acetate (50 mL), filtered through a short plug of Celite, and washed with H 2 O (50 mL) and brine. The organic layer was combined, dried over Na 2 SO 4 , filtered, and then concentrated under reduced pressure. The crude product was purified by flash column chromatography. Difluoromethyl-arylations of alkenes In a nitrogen-filled glovebox, a 4 mL vial equipped with a stir bar was charged with [Cu(MeCN) 4 ]BF 4 (20 mol%, 15.5 mg), terpyridine ( L1 ) (20 mol%, 11.8 mg), alkenes (0.75 mmol, 3.0 equiv. ), and 200 μL DMSO. A solution of diazonium salts (0.25 mmol, 1.0 equiv.) in 400 μL DMSO, and a solution of (DMPU) 2 Zn(CF 2 H) 2 (0.2 mmol, 87 mg, 0.8 equiv.) in 400 μL DMSO were slowly added to the vial with syringes at the same time over the course of 10 min. The resultant mixture was stirred at room temperature for 30 min. After the reaction was completed, the mixture was diluted with ethyl acetate (50 mL), filtered through a short plug of Celite, and washed with H 2 O (50 mL) and brine. The organic layer was combined, dried over Na 2 SO 4 , filtered, and then concentrated under reduced pressure. The crude product was purified by flash column chromatography.